Dendritic cell subsets require cis-activation for cytotoxic CD8 T-cell induction Dendritic cells (DCs) are required for the induction of cytotoxic T cells (CTL). In most tissues, including the lung, the resident DCs fall into two types expressing the integrin markers CD103 and CD11b. The current supposition is that DC function is predetermined by lineage, designating the CD103 + DC as the major cross-presenting DC able to induce CTL. Here we show that Poly I:C (TLR3 agonist) or R848 (TLR7 agonist) do not activate all endogenous DCs. CD11b + DCs can orchestrate a CTL response in vivo in the presence of a TLR7 agonist but not a TLR3 agonist, whereas CD103 + DCs require ligation of TLR3 for this purpose. This selectivity does not extend to antigen cross-presentation for T-cell proliferation but is required for induction of cytotoxicity. Thus, we demonstrate that the ability of DCs to induce functional CTLs is specific to the nature of the pathogen-associated molecular pattern (PAMP) encountered by endogenous DC. Dendritic cells (DCs) are professional antigen-presenting cells with the capacity to acquire antigen, migrate to the draining lymph node (LN) and initiate T-cell-mediated immunity. Tissue-resident DCs are heterogeneous and functionally diverse. DCs differ in their expression of surface integrins, pattern recognition receptors (PRR), transcriptional regulation and antigen-presentation capabilities [1] , [2] , [3] , [4] , [5] , [6] , [7] . In the lung, there are two DC populations, which are identified by the integrins they highly express, CD103 + DCs and CD11b + DCs. Both subsets are referred to as migratory DCs since they migrate to the draining LN and present antigen to T cells. These DCs uniquely express Toll-like receptors (TLRs): TLR3 by CD103 + DCs and TLR7 by CD11b + DCs [7] . These two TLRs are both endosomal viral nucleic acid sensors that recognize double-stranded RNA (dsRNA) and single-stranded RNA, respectively, and both TLR3 and TLR7 agonists are known to be highly effective in generating protective T-cell-mediated immunity. Subsequently, this has led to the presumption that viral nucleic acids stimulate all DCs found in tissue, ultimately resulting in an effector T-cell response. Here we sought to determine how these pathogen-associated molecular patterns (PAMPs; TLR3 and TLR7 agonists) in vivo activate DC subsets in the lung. We hypothesized that both pulmonary DC subsets can induce a cytotoxic T-cell (CTL) response but that only one pulmonary DC subset is activated in the presence of either Poly I:C (TLR3 ligand) or R848 (TLR7 ligand) to induce CTL. Data supporting our hypothesis were based on ex vivo analysis or within bone marrow-derived chimeric mice that showed TLRs need to be ligated directly on the DC to induce a CTL response [8] , [9] , [10] , [11] , [12] , [13] , [14] , and that the presence of an inflammatory milieu alone does not drive the process of T-cell differentiation [13] , [14] . However, it remains unclear how TLR3 and TLR7 agonists activate endogenous DC subsets in vivo , and which subset is responsible for generating protective T-cell-mediated immunity in the presence of these TLR agonists. DCs have the capacity to present exogenous antigens as peptides on major histocompatibility complex (MHC) class I (cross-presentation), which are recognized by antigen-specific CD8 T cells. Subsequently, depending on the activation status of the antigen-presenting DCs, proliferating antigen-specific CD8 T cells can be instructed to develop into CTLs [15] , [16] . In this study, we use proliferation of antigen-specific CD8 T cells as a readout of antigen cross-presentation by DCs, and an in vivo killing assay as a readout of T-cell cytotoxic function. We and others have previously demonstrated the unique ability of CD103 + DCs to take up apoptotic cells, migrate to the LNs and cross-present cell-associated antigens to CD8 T cells in vivo [7] , [17] , [18] , [19] , [20] . Moreover, in the presence of TLR3 agonists, the combination of CD103 + DC uptake of apoptotic cells, activation and antigen cross-presentation resulted not only in CD8 T-cell proliferation but also in the subsequent differentiation of CTL [7] . In turn, most studies have suggested that CD103 + DCs are the dominant cross-presenting DCs in the lung [6] , [7] , [17] , [21] , [22] , [23] . In contrast, CD11b + DCs have been thought to mainly present exogenous antigen via MHC II to CD4 T cells [6] , [7] , [24] , [25] , [26] . However, in this study, we demonstrate within a primary immune response that both DC subsets in the lung have the capacity to induce antigen-specific CTL, but only if they are simultaneously (1) able to acquire and present the antigen, and (2) are activated through their corresponding PRR (referred to as matched; Supplementary Fig. 1 ). Thus, if the antigen-presenting DC-TLR agonist pair is mismatched in that the DCs are either (1) presenting the antigen but not stimulated by their corresponding TLR agonist, or (2) activated by their corresponding TLR agonist but not presenting the antigen, then an antigen-specific CTL responses will not occur. Induction of CTL has long been known to be critical for controlling infections and tumorigenesis, and here we report how each DC subset in the lung can function to promote such responses. CD11b + DCs induce CTL in the presence of a TLR7 agonist Microarray analysis was performed to identify PRR candidates that selectively activate individual DC subsets to induce CTL. At the mRNA level, the most striking expressional difference between the two DC subsets was TLR3 by CD103 + DCs and TLR7 by CD11b + DCs ( Fig. 1a ) [7] . Based on this disparity, we hypothesized that Poly I:C, a TLR3 agonist, would solely activate TLR3-expressing CD103 + DC, and not CD11b + DCs, to induce CTL; whereas R848, a TLR7 agonist, would activate TLR7-expressing CD11b + DCs, but not CD103 + DC, to induce CTL. To address this hypothesis, we first identified migratory DCs in the lung and lung-draining LN (LLN) as CD11c + and MHCII hi ( Fig. 1b and Supplementary Fig. 2a ). Wild-type (WT) mice displayed both migratory CD103 + and CD11b + DCs. In contrast, Batf3 −/− mice, deficient for the Batf3 transcription factor and lacking CD103 + DCs, only had CD11b + DCs ( Fig. 1b and Supplementary Fig. 2a ) [7] , [21] . To exclusively target soluble antigen to CD11b + DCs, soluble OVA (sOVA) was instilled intranasally (i.n.) into Batf3 −/− mice, thereby allowing transportation of antigen solely by CD11b + DCs to the LLN ( Fig. 1c and Supplementary Fig. 2b ) [4] , [6] , [7] , [27] . 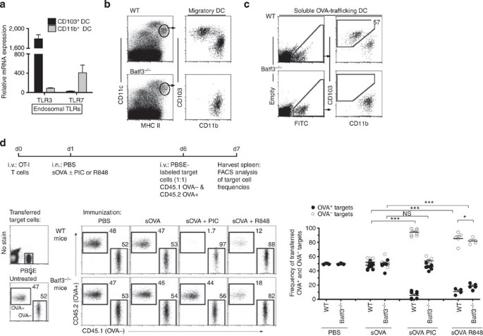Figure 1: CD11b+DCs induce CTLs in the presence of a TLR7 agonist. (a) Pulmonary DCs were isolated for microarray analysis. Bar graph shows relative mRNA expression of the indicated genes for CD103+DCs (black) and CD11b+DCs (grey). Error bars represent s.e.m.,n=3. (b) Gating of migratory CD11c+MHCIIhiDCs in the lung-draining LN (LLN) of WT and Batf3−/−mice. (c) LLN 24 h post i.n. delivery of FITC-labelled sOVA. Left, live cells plotted as empty channel (no stain) versus FITC to identify antigen-bearing FITC+cells. Right, antigen-bearing DCs plotted as CD103 versus CD11b to display the antigen+DCs present in the LLN. (d) Top, experimental setup. OT-I cells (1 × 106total cells) were transferred into WT and Batf3−/−mice 1 day before i.n. immunization with PBS or 1 μg sOVA+/−10 μg Poly I:C (PIC) or 50 μg R848. Five days later, mice were i.v. injected with (1:1) PBSE-labelled OVA−(CD45.1+) and OVA+(CD45.2+) target cells. Twenty-four hours post-target cell transfer, cytotoxicity was assessed by flow cytometry. Dot plots display the frequencies of transferred target cells: OVA−(open) versus OVA+(closed) cells. Each dot represents one mouse. Data are representative of at least four independent experiments with 3–4 mice per group. ***P<0.0001, *P<0.03,t-test. NS, not significant. Figure 1: CD11b + DCs induce CTLs in the presence of a TLR7 agonist. ( a ) Pulmonary DCs were isolated for microarray analysis. Bar graph shows relative mRNA expression of the indicated genes for CD103 + DCs (black) and CD11b + DCs (grey). Error bars represent s.e.m., n =3. ( b ) Gating of migratory CD11c + MHCII hi DCs in the lung-draining LN (LLN) of WT and Batf3 −/− mice. ( c ) LLN 24 h post i.n. delivery of FITC-labelled sOVA. Left, live cells plotted as empty channel (no stain) versus FITC to identify antigen-bearing FITC + cells. Right, antigen-bearing DCs plotted as CD103 versus CD11b to display the antigen + DCs present in the LLN. ( d ) Top, experimental setup. OT-I cells (1 × 10 6 total cells) were transferred into WT and Batf3 −/− mice 1 day before i.n. immunization with PBS or 1 μg sOVA +/− 10 μg Poly I:C (PIC) or 50 μg R848. Five days later, mice were i.v. injected with (1:1) PBSE-labelled OVA − (CD45.1 + ) and OVA + (CD45.2 + ) target cells. Twenty-four hours post-target cell transfer, cytotoxicity was assessed by flow cytometry. Dot plots display the frequencies of transferred target cells: OVA − (open) versus OVA + (closed) cells. Each dot represents one mouse. Data are representative of at least four independent experiments with 3–4 mice per group. *** P <0.0001, * P <0.03, t -test. NS, not significant. Full size image In order to determine whether TLR agonists selectively activate individual DC subsets to induce a CTL response against soluble antigen, we used an in vivo CTL killing assay (schematic outline, Fig. 1d ). First, OVA-specific CD8 + T cells (OT-I T cells) were adoptively transferred into WT and Batf3 −/− mice. One day later, sOVA (trafficked by both migratory DC subsets in WT mice and only CD11b + DCs in Batf3 −/− mice; Fig. 1c ) was instilled i.n. with phosphate-buffered saline (PBS), 10 μg Poly I:C or 50 μg R848. Five days post antigen delivery, (Pacific blue succinimidyl ester) PBSE-labelled target cells, CD45.1 WT (OVA − ) and CD45.2 OVA-expressing (OVA + ) splenocytes, were intravenously (i.v.) delivered at a 1:1 ratio for the measurement of antigen-specific killing. Twenty-four hours after target cell delivery, in vivo CTL responses were assessed by measuring the killing of OVA + target cells compared with OVA − target cells ( Fig. 1d ). Following immunization with PBS or sOVA alone, the spleens of WT and Batf3 −/− mice contained equal ratios of OVA + and OVA − target cells ( Fig. 1d ), indicating a lack of CTL responses. In contrast, immunization with sOVA and Poly I:C resulted in selective killing of OVA + CD45.2 target cells in WT mice. Strikingly, OVA-specific killing was absent in Batf3 −/− mice (which lack TLR3-expressing CD103 + DCs). These data suggest that of the two migrating DC subsets, only CD103 + DCs have the capacity to recognize and respond to Poly I:C by inducing a CTL response. To ascertain whether the TLR7-expressing CD11b + DCs were functionally capable of inducing a CTL response in the Batf3 −/− mice, the in vivo CTL assay was repeated using sOVA and a TLR7 agonist, R848 ( Fig. 1d ). Notably, in the presence of a TLR7 agonist, both WT and Batf3 −/− mice demonstrated killing of OVA + target cells. Thus, in the absence of CD103 + DCs, CD11b + DCs could induce CTL. These data indicate that CD11b + DCs are in fact capable of inducing CTL when stimulated with R848 but not Poly I:C. The lack of antigen-specific CTL in Batf3 −/− mice treated with sOVA and Poly I:C was not due to the lack of proliferating antigen-specific T cells. Both pulmonary DCs cross-presented OVA as detected by OVA-SIINFEKL peptide on MHC I, resulting in the proliferation of OT-I T cells in both WT and Batf3 −/− mice ( Fig. 2a and Supplementary Fig. 3a ). The proliferation of OT-I T cells was independent of Poly I:C ( Fig. 2a ). Even though antigen-specific CD8 T-cell proliferation occurred in the Batf3 −/− mice, the extent of carboxyfluorescein succinimidyl ester (CFSE) dilution was lower compared with WT mice, indicating that fewer CD8 T cells have undergone the final rounds of division ( Fig. 2a ). In the Batf3 −/− mice, the overall impaired proliferation of antigen-specific CD8 T cells could indicate diminished activation of antigen-presenting CD11b + DCs without an added adjuvant (TLR ligand). Alternatively, reduced antigen-specific CD8 T-cell proliferation in Batf3 −/− mice could reflect the reduced number of trafficking pulmonary DCs available to present antigen, which are only half of the normal migratory DCs found in the LLNs of WT mice ( Fig. 2a ) [7] , [21] . Therefore, we sought to determine whether the lack of OVA + target killing in Batf3 −/− mice ( Fig. 1d ) was due to fewer CD8 T-cell numbers or a deficiency in T-cell function. To assess T-cell function from OVA-immunized WT and Baft3 −/− mice, OT-I CD8 T cells were extracted from immunized WT and Batf3 −/− mice, transferred in equal numbers into naive WT recipients and examined for cytotoxic function in these new hosts ( Fig. 2b ). To do this, CD45.1 OT-I T cells were adoptively transferred into CD45.2 WT and CD45.2 Batf3 −/− mice. Twenty-four hours later, the animals were immunized with sOVA and Poly I:C. Five days later, the responding CD45.1 OT-I T cells were isolated from the spleens, purified and adoptively transferred into naive WT mice, which 24 h after received a 1:1 ratio of PBSE-labelled OVA − and OVA + target cells to assess cytotoxicity ( Fig. 2b ). When equal numbers of proliferating OT-I T cells were transferred into naive WT mice, differentiated OT-I T cells from WT mice, but not Batf3 −/− mice, displayed cytotoxic function ( Fig. 2b ). Based on these data, the lack of CTL in Batf3 −/− mice immunized with OVA + Poly I:C cannot be attributed to either the lack of antigen presentation by CD11b + DCs or a decrease in proliferating antigen-specific T cells. Instead, the absence of CD103 + DCs in the Batf3 −/− mice immunized with OVA + Poly I:C resulted in the proliferation of antigen-specific T cells lacking cytotoxic function. Furthermore, owing to the high frequency of adoptively transferred OVA-specific T cells, we investigated whether Batf3 −/− mice could cross-present OVA to endogenous T cells. We observed the accumulation of H-2Kb/SIINFEKL tetramer + T cells in the LLNs of both WT and Batf3 −/− mice 4 days after immunization with OVA and Poly I:C ( Supplementary Fig. 3b ). Overall, these data demonstrate that antigen-specific CD8 T-cell proliferation occurs independently of TLR3 signalling by the cross-presenting CD103 + DCs ( Supplementary Fig. 4 ). 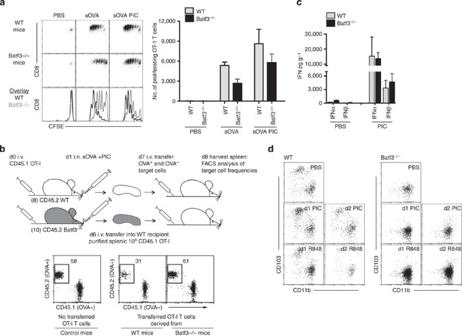Figure 2: Mice deficient of TLR3+CD103+DCs cannot induce antigen-specific CTLs in the presence of Poly I:C (PIC). (a) CFSE-labelled OT-I CD8 T cells (1 × 106total cells) were adoptively transferred into WT and Batf3−/−mice 1 day before i.n. delivery of PBS or 1 μg sOVA±10 μg PIC. T-cell proliferation was assessed 3 days later by FACS (left). Bar graphs show total numbers of proliferating OT-I CD8 T cells (right). Data are representative of three independent experiments of three mice per group. (b) CD45.1+OT-I CD8 T cells were adoptively transferred into WT and Batf3−/−mice 1 day before i.n. delivery of 1 μg sOVA+10 μg PIC. Five days after instillation, CD45.1+OT-I CD8 T cells were purified from spleens of 8 WT and 10 Batf3−/−mice. CD45.1+OT-I CD8 T cells (1 × 106) purified from either WT or Batf3−/−mice were adoptively transferred into naive WT mice. Twenty-four hours later, PBSE-labelled OVA−and OVA+target cells were transferred. Twenty-four hours later, spleens were assessed for target cell frequency. Data shown is a representative experiment of two independent experiments of four mice per group. (c) By enzyme-linked immunosorbent assay, type I IFNs were detected in the lungs of WT and Baft3−/−mice 10 h after i.n. delivery of PBS or 10 μg PIC. Error bars, s.e.m. Data shown is a representative experiment of two independent experiments with five mice per group. (d) In the LLN, migratory DCs were analysed in WT and Batf3−/−mice for the presence of CD103+DCs 1 and 2 days after i.n. delivery of 10 μg PIC or 50 μg R848. CD11c+MHCIIhiLy6C-migratory DCs were plotted as CD103 versus CD11b. Data shown is a representative experiment of two independent experiments. Figure 2: Mice deficient of TLR3 + CD103 + DCs cannot induce antigen-specific CTLs in the presence of Poly I:C (PIC). ( a ) CFSE-labelled OT-I CD8 T cells (1 × 10 6 total cells) were adoptively transferred into WT and Batf3 −/− mice 1 day before i.n. delivery of PBS or 1 μg sOVA±10 μg PIC. T-cell proliferation was assessed 3 days later by FACS (left). Bar graphs show total numbers of proliferating OT-I CD8 T cells (right). Data are representative of three independent experiments of three mice per group. ( b ) CD45.1 + OT-I CD8 T cells were adoptively transferred into WT and Batf3 −/− mice 1 day before i.n. delivery of 1 μg sOVA+10 μg PIC. Five days after instillation, CD45.1 + OT-I CD8 T cells were purified from spleens of 8 WT and 10 Batf3 −/− mice. CD45.1 + OT-I CD8 T cells (1 × 10 6 ) purified from either WT or Batf3 −/− mice were adoptively transferred into naive WT mice. Twenty-four hours later, PBSE-labelled OVA − and OVA + target cells were transferred. Twenty-four hours later, spleens were assessed for target cell frequency. Data shown is a representative experiment of two independent experiments of four mice per group. ( c ) By enzyme-linked immunosorbent assay, type I IFNs were detected in the lungs of WT and Baft3 −/− mice 10 h after i.n. delivery of PBS or 10 μg PIC. Error bars, s.e.m. Data shown is a representative experiment of two independent experiments with five mice per group. ( d ) In the LLN, migratory DCs were analysed in WT and Batf3 −/− mice for the presence of CD103 + DCs 1 and 2 days after i.n. delivery of 10 μg PIC or 50 μg R848. CD11c + MHCII hi Ly6C - migratory DCs were plotted as CD103 versus CD11b. Data shown is a representative experiment of two independent experiments. Full size image Since type 1 interferons (IFN) are key cytokines critical for CTL responses, we examined whether Batf3 −/− mice lacked type 1 IFN production in the presence of Poly I:C. We observed equivalent levels of type 1 IFNs in the lungs of both WT and Batf3 −/− mice instilled with 10 μg of Poly I:C, suggesting that type 1 IFNs alone were not sufficient to activate antigen-bearing DCs to induce CTL ( Fig. 2c ) [13] , [14] . To ensure that CD11b + DCs were the antigen-presenting cells driving the induction of CTL after instillation with R848, other known TLR7-expressing myeloid cells were depleted. Anti-Gr1 antibody (recognizing both Ly6C and Ly6G) was used to deplete TLR7-expressing monocytes and plasmacytoid DCs [28] , [29] . Regardless of the presence or absence of monocytes and plasmacytoid DCs in WT and Batf3 −/− mice, the induction of CTL following the administration of R848 was similar, suggesting that pulmonary CD11b + DCs were the primary inducers of CTL in the LLNs ( Supplementary Fig. 5 ). It has been reported that during infection or treatment with interleukin (IL)-12, CD103 + DCs can develop in Batf3 −/− mice [30] . Therefore, to ensure that CD11b + DCs, and not the return of CD103 + DCs, account for the induction of CTL in Batf3 −/− mice immunized with R848, we examined whether the instillation of 50 μg R848 resulted in the development of CD103 + DCs. In our experimental model, one i.n. dose of either 10 μg Poly I:C or 50 μg R848 did not result in the development of CD103 + DCs in Batf3 −/− mice ( Fig. 2d ). Overall these data support that antigen-bearing CD11b + DCs, stimulated by R848, can induce CTL. R848 does not activate antigen-bearing CD103 + DC to induce CTL To further confirm that CTL induction by antigen-bearing DCs requires direct ligation of their TLR, antigen-bearing CD103 + DCs were investigated for their capacity to induce CTL in the presence of TLR3 agonist, Poly I:C (matched) or TLR7 agonist, R848 (mismatched). To demonstrate exclusive targeting of antigen to CD103 + DCs, CFSE-labelled OVA-expressing apoptotic cells were instilled ( Fig. 3a ) [7] . As previously shown, CD103 + DCs were the sole carriers and presenters of cell-associated antigens in the LLN. This was confirmed in Batf3 −/− mice, in which apoptotic cell-associated antigens were unable to be transported or presented owing to their lack of CD103 + DCs ( Fig. 3a ) [7] . The selectivity of apoptotic cell acquisition by CD103 + DC is potentially because of the selective expression of multiple phosphatidylserine receptors compared with CD11b + DCs [7] . Overall, the uptake of apoptotic cells represents a specialized form of phagocytosis (more closely related to stimulated macropinocytosis), and requires both a tethering (that is, recognition) step as well as a Rac-dependent uptake process [31] . 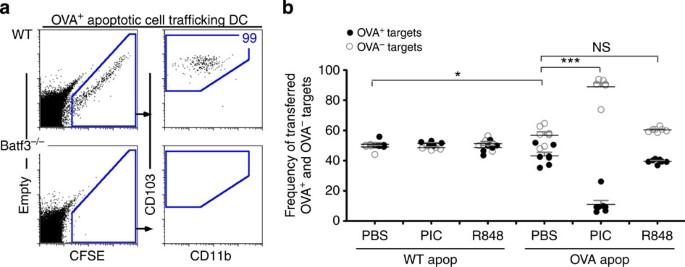Figure 3: Antigen-bearing DC require matched TLR agonist to induce CTL. (a) FACS analysis of cells within the LLN 24 h post i.n. delivery of CFSE-labelled OVA+apoptotic (apop) thymocytes. Left, live cells plotted as empty channel (no stain) versus CFSE to identify antigen-bearing CFSE+cells. Right, antigen-bearing DCs plotted as CD103 versus CD11b to display the antigen+DCs in the LLN. (b) OT-I CD8 T cells were adoptively transferred into WT mice 1 day before i.n. instillation of WT (OVA−) or OVA+apoptotic cells±10 μg Poly I:C (PIC) or 50 μg R848. Five days after apoptotic cell administration, PBSE-labelled OVA−and OVA+target cells were transferred. Twenty-four hours later, spleens were assessed for target cell frequency. Each dot represents one mouse. ***P<0.0001, *P<0.02,t-test. NS, non-significant. Figure 3: Antigen-bearing DC require matched TLR agonist to induce CTL. ( a ) FACS analysis of cells within the LLN 24 h post i.n. delivery of CFSE-labelled OVA + apoptotic (apop) thymocytes. Left, live cells plotted as empty channel (no stain) versus CFSE to identify antigen-bearing CFSE + cells. Right, antigen-bearing DCs plotted as CD103 versus CD11b to display the antigen + DCs in the LLN. ( b ) OT-I CD8 T cells were adoptively transferred into WT mice 1 day before i.n. instillation of WT (OVA − ) or OVA + apoptotic cells±10 μg Poly I:C (PIC) or 50 μg R848. Five days after apoptotic cell administration, PBSE-labelled OVA − and OVA + target cells were transferred. Twenty-four hours later, spleens were assessed for target cell frequency. Each dot represents one mouse. *** P <0.0001, * P <0.02, t -test. NS, non-significant. Full size image I.n. delivery of OVA-expressing apoptotic cells with Poly I:C led to robust antigen-specific killing, that is, the TLR agonist directly activated the antigen-bearing CD103 + DC ( Fig. 3b ) [7] , [32] . On the other hand, when OVA-expressing apoptotic cells were instilled in the presence of R848, there was no additional killing above the observed background cytotoxicity in mice immunized with OVA-expressing apoptotic cells alone ( Fig. 3b ), and only a minor accumulation of IFNγ in the proliferating T cells ( Supplementary Fig. 6 ). As controls, administration of WT (OVA − ) apoptotic cells with Poly I:C or R848 did not result in killing of OVA + target cells. These data demonstrate that a TLR7 agonist could not activate the antigen-bearing TLR3 + CD103 + DC to induce CTL. Thus, supporting the concept that antigen-bearing DCs require direct stimulation of their expressed PRRs to induce CTL. Cell-associated and soluble antigens are processed differently in CD103 + DCs Since pulmonary CD103 + DCs exhibited the greatest level of TLR3 protein among all haematopoietic and non-haematopoietic cells in the lung ( Fig. 4a and Supplementary Fig. 7 ), we sought to determine whether TLR3 was required for the activation of CD103 + DCs by Poly I:C in an in vivo CTL assay (as in Fig. 1d ). In contrast to WT mice, i.n. delivery of OVA-expressing apoptotic cells with Poly I:C did not lead to antigen-specific killing of OVA + target cells in TLR3 −/− mice ( Fig. 4b ). The lack of CTL differentiation in the TLR3 −/− mice was not due to diminished antigen-specific T-cell proliferation, as revealed by pronounced OT-I T-cell division in both WT and TLR3 −/− mice ( Fig. 4c ). Taken together, these data suggest that ligation of TLR3 is required to activate CD103 + DCs to induce antigen-specific CTL but not T-cell proliferation. 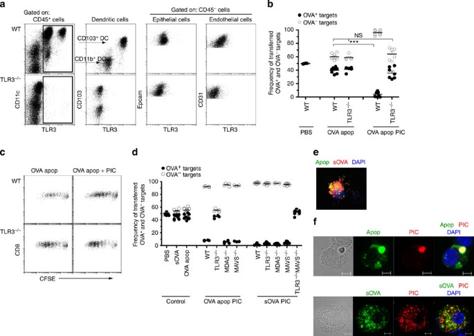Figure 4: Cell-associated and soluble antigens are processed differently in CD103+DCs. (a) TLR3 protein expression of haematopoietic (CD45+) and non-haematopoietic (CD45−) cells isolated from the lungs of WT and TLR3−/−mice. DCs were identified as low SSC CD11c+MHCIIhicells before being plotted as CD103 versus TLR3. (b,d) OT-I CD8 T cells were adoptively transferred into WT, TLR3−/−, MDA5−/−, MAVS−/−or TLR3−/−MAVS−/−mice 1 day before i.n. delivery of PBS, sOVA or OVA+apoptotic (apop) cells±10 μg Poly I:C (PIC). Five days after immunization, mice were given PBSE-labelled target (OVA−or OVA+) cells. Twenty-four hours later, spleens were assessed for target cell frequency. Each dot represents one mouse. Data represent at least three independent experiments with 3–4 mice per group. ***P<0.0001t-test. (c) CFSE-labelled OT-I CD8 T cells (1 × 106total cells) were adoptively transferred into WT and TLR3−/−mice 1 day before i.n. delivery of OVA+apoptotic cells±10 μg PIC. T-cell proliferation was assessed 3 days later by FACS. (e) Microscopy analysis of isolated pulmonary CD103+DCs 2 h after i.n. co-delivery of CFSE-labelled apoptotic cells (green) and sOVA-Alexa 647 (red) and DAPI (blue). (f) Microscopy analysis of isolated pulmonary CD103+DCs 2 h after i.n. co-delivery of CFSE-labelled apoptotic cell (green) or sOVA-FITC (green) with rhodamine-labelled PIC (red) and DAPI (blue). Scale bars, 5 μm. Data represent at least four independent experiments with 10–20 CD103+antigen-bearing DCs analysed per slide. Figure 4: Cell-associated and soluble antigens are processed differently in CD103 + DCs. ( a ) TLR3 protein expression of haematopoietic (CD45 + ) and non-haematopoietic (CD45 − ) cells isolated from the lungs of WT and TLR3 −/− mice. DCs were identified as low SSC CD11c + MHCII hi cells before being plotted as CD103 versus TLR3. ( b , d ) OT-I CD8 T cells were adoptively transferred into WT, TLR3 −/− , MDA5 −/− , MAVS −/− or TLR3 −/− MAVS −/− mice 1 day before i.n. delivery of PBS, sOVA or OVA + apoptotic (apop) cells±10 μg Poly I:C (PIC). Five days after immunization, mice were given PBSE-labelled target (OVA − or OVA + ) cells. Twenty-four hours later, spleens were assessed for target cell frequency. Each dot represents one mouse. Data represent at least three independent experiments with 3–4 mice per group. *** P <0.0001 t -test. ( c ) CFSE-labelled OT-I CD8 T cells (1 × 10 6 total cells) were adoptively transferred into WT and TLR3 −/− mice 1 day before i.n. delivery of OVA + apoptotic cells±10 μg PIC. T-cell proliferation was assessed 3 days later by FACS. ( e ) Microscopy analysis of isolated pulmonary CD103 + DCs 2 h after i.n. co-delivery of CFSE-labelled apoptotic cells (green) and sOVA-Alexa 647 (red) and DAPI (blue). ( f ) Microscopy analysis of isolated pulmonary CD103 + DCs 2 h after i.n. co-delivery of CFSE-labelled apoptotic cell (green) or sOVA-FITC (green) with rhodamine-labelled PIC (red) and DAPI (blue). Scale bars, 5 μm. Data represent at least four independent experiments with 10–20 CD103 + antigen-bearing DCs analysed per slide. Full size image In contrast to cell-associated antigen, when the requirement of TLR3 was examined in mice that received soluble antigen and Poly I:C, a different result was observed; CTL was induced in WT and TLR3 −/− mice immunized with sOVA and Poly I:C ( Fig. 4d ). Since the presence of CD103 + DCs was required for the induction of CTL upon immunization with Poly I:C (Batf3 −/− mice have no CTL in the presence of Poly I:C; Fig. 1b ) and TLR3 was dispensable when Poly I:C was delivered with soluble antigen, the role of other dsRNAs sensors was investigated. In addition to endosomal TLR3, Poly I:C could bind cytosolic dsRNA sensors such as MDA5 and RIG-I, both of which commonly signal through MAVS [33] . To test the contribution of dsRNA cytosolic sensors, MDA5 −/− or MAVS −/− mice were immunized with sOVA and Poly I:C and displayed similar CTL responses as WT mice ( Fig. 4d ). The complete killing of OVA + target cells in these mice raised the possibility that in the case of soluble antigen, both endosomal and cytosolic dsRNA sensors are utilized by CD103 + DCs for the detection of Poly I:C and subsequent activation of CTL. To address this possibility, we bred TLR3 −/− MAVS −/− mice and performed the in vivo CTL assay using sOVA and Poly I:C. TLR3 −/− MAVS −/− mice displayed complete abrogation of CTL responses compared with WT, TLR3 −/− , MDA5 −/− and MAVS −/− mice ( Fig. 4d ). These data suggest that soluble antigen and Poly I:C can utilize either the endosomal or cytosolic dsRNA-sensing pathways ( Fig. 4d ), whereas cell-associated antigens in the presence of Poly I:C require the TLR3 endosomal pathways ( Fig. 4b,d ). Furthermore, when the physical location of cell-associated antigen and sOVA were examined by microscopy within CD103 + DCs, cell-associated antigen was found solely in endosomal vesicles, whereas sOVA was found within the endosomal and cytosolic compartments ( Fig. 4e ). In addition, delivery of Poly I:C with cell-associated antigen resulted in the colocalization of Poly I:C and antigen within the same endosomal vesicles, whereas delivery of Poly I:C with sOVA was detected in both endosomal and cytosolic compartments ( Fig. 4f ). Thus, the physical nature of the antigen may dictate the mode of dsRNA sensing by CD103 + DCs. TLR7 ligation enables CD11b + DCs to induce CTL Next, we examined whether TLR7 was required to activate antigen-bearing CD11b + DCs to induce antigen-specific CTL. Indeed compared with WT mice, TLR7 −/− mice given sOVA and R848 failed to elicit substantial antigen-specific killing of OVA + target cells in vivo ( Fig. 5a ). As controls, WT and TLR7 −/− mice immunized with sOVA and Poly I:C mounted a robust CTL response. Thus, unlike Poly I:C, which could signal through multiple PRRs in the context of soluble antigen, TLR7 ligation by R848 appeared essential to activate CD11b + DCs to induce CTL. 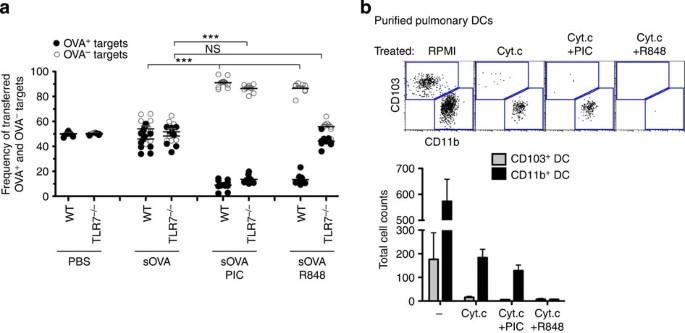Figure 5: TLR7 ligation is required for CD11b+DCs to induce CTL. (a) OT-I CD8 T cells were adoptively transferred into WT or TLR7−/−, mice 1 day before i.n. delivery of PBS, sOVA±10 μg Poly I:C (PIC) or 50 μg R848. Five days after immunization, mice were given PBSE-labelled target (OVA−or OVA+) cells. Twenty-four hours later, spleens were assessed for target cell frequency. Each dot represents one mouse. Data represent at least three independent experiments with 3–4 mice per group. ***P<0.0001,t-test. (b) Enriched CD11c+cells from the lung were plated overnight in triplicate±10 mg ml−1horse cytochromec(Cyt.c) with 10 μg ml−1PIC or 50 μg ml−1R848. FACS plots show ratios of isolated DAPI−MHC II+DCs (upper) and total DC cell counts (below). Data are representative of three independent experiments. NS, non-significant. Figure 5: TLR7 ligation is required for CD11b + DCs to induce CTL. ( a ) OT-I CD8 T cells were adoptively transferred into WT or TLR7 −/− , mice 1 day before i.n. delivery of PBS, sOVA±10 μg Poly I:C (PIC) or 50 μg R848. Five days after immunization, mice were given PBSE-labelled target (OVA − or OVA + ) cells. Twenty-four hours later, spleens were assessed for target cell frequency. Each dot represents one mouse. Data represent at least three independent experiments with 3–4 mice per group. *** P <0.0001, t -test. ( b ) Enriched CD11c + cells from the lung were plated overnight in triplicate±10 mg ml −1 horse cytochrome c (Cyt. c ) with 10 μg ml −1 PIC or 50 μg ml −1 R848. FACS plots show ratios of isolated DAPI − MHC II + DCs (upper) and total DC cell counts (below). Data are representative of three independent experiments. NS, non-significant. Full size image A unique function of splenic CD8 + DCs is their ability to release endosomal contents into the cytosol as a mechanism for proteasome-dependent cross-presentation [34] , [35] . This phenomenon was demonstrated by i.v. injecting cytochrome c into mice, which resulted in the selective elimination of splenic CD8a + DCs via activation of apoptosis when cytochrome c was released into the cytosol from the endosomal compartment [36] . Therefore, using an ex vivo adaptation of this system, we investigated whether CD103 + or CD11b + DCs shared this antigen-processing feature. In overnight culture, cytochrome c alone induced apoptosis of pulmonary CD103 + DCs, which share similar functional properties with splenic CD8 + DCs ( Fig. 5b ). CD11b + DCs were less susceptible to cytochrome c -induced apoptosis, although some effects were seen. Next, we determined whether TLR7 ligation of CD11b + DCs could mediate enhanced release of endosomal content into the cytosol. While the addition of Poly I:C to cytochrome c had little effect on the apoptosis of CD11b + DCs in culture compared with cytochrome c alone, R848 added along with cytochrome c completely ablated CD11b + DCs in culture. This was presumably due to enhanced release of cytochrome c into the cytosol ( Fig. 5b ). These data suggest that the background killing observed in CD11b + DCs cultured with cytochrome c alone may account for the cross-presentation observed in the Batf3 −/− mice in the absence of added TLR ligand ( Fig. 2a ). However, the addition of R848 to the cytochrome c culture rendered CD11b + DCs more susceptible to apoptosis, which seemed to parallel with enhanced cross-presentation (indirectly measured by antigen-specific CD8 T-cell proliferation) in Batf3 −/− mice immunized with sOVA and R848 ( Supplementary Fig. 8 ). Thus, the ligation of TLR7 on CD11b + DCs may alter how CD11b + DCs process endosomal cargo by triggering the release of endosomal contents into the cytosol for enhanced antigen-specific T-cell proliferation and induction of CTL ( Fig. 1d and Supplementary Fig. 8 ). IL-27 is a key mediator for the induction of CTL The differentiation of a naive T cell into an effector T cell requires signal 1 (TCR:MHC), signal 2 (co-stimulatory molecules) and signal 3 (cytokine stimulation) from an antigen-presenting cell. Studies have demonstrated that the intensity of signal 2 (based on the expression of co-stimulatory molecules such as CD40, CD80 and CD86) on migratory DCs does not necessarily determine whether the DC promotes tolerance or immunity [37] . Therefore, we investigated the role of cytokines, signal 3, produced by the antigen-bearing DCs for the induction of CTL. Since different PAMPs disparately activate the two pulmonary DC subsets to induce CTL, we investigated by microarray analysis the changes in cytokine expression by activated pulmonary DCs that were stimulated with either Poly I:C or R848. At the gene level, IL-12 and IL-27 were selectively expressed by Poly I:C-activated CD103 + DCs and R848-activated CD11b + DCs ( Fig. 6a ). In addition, the selective expression of IL-12 by activated pulmonary DCs was confirmed using IL-12p40 reporter mice ( Fig. 6b ). These findings led us to examine the contribution of IL-12 and IL-27 for the induction of CTL. Using the in vivo CTL assay, WT, IL-12 −/− and IL-27 −/− mice were immunized with OVA + apoptotic cells (only presented by CD103 + DCs) along with Poly I:C. Both WT and IL-12 −/− mice had robust CTL responses, whereas IL-27 −/− mice displayed reduced cytotoxicity, indicating that IL-27, but not IL-12, contributed to the induction of CTL ( Fig. 6c ). A similar outcome was observed when WT, IL-12 −/− and IL-27 −/− mice were immunized with sOVA (presented by both migratory DCs) and Poly I:C or R848. However, since it is possible that IL-27 may compensate for the lack of IL-12 in IL-12 −/− mice, double knockout mice were created to definitively prove that IL-12 does not substantially contribute to the induction of CTL. 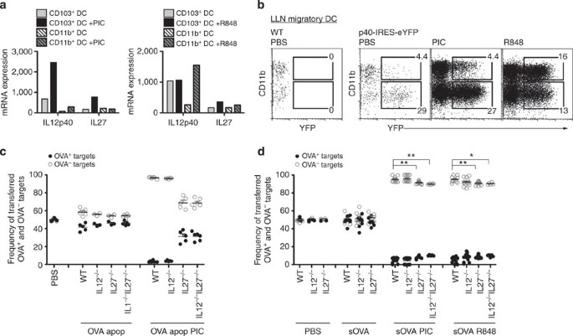Figure 6: IL-27 and not IL-12 is a key mediator for the induction of CTL. (a) DC subsets were isolated from PBS-perfused lung tissue for microarray analysis. Bars show relative mRNA expression of the indicated genes in pulmonary CD103+DCs and CD11b+DCs treated± PIC or R848. (b) FACS analysis of migratory DCs isolated from LLN of IL-12p40 reporter mice, 24 h post i.n. instillation of 10 μg Poly I:C (PIC) or 50 μg R848. (c,d) OT-I CD8 T cells were adoptively transferred into WT, IL-12−/−, IL-27−/−or IL-12−/−IL-27−/−mice 1 day before i.n. delivery of PBS, sOVA or OVA+apoptotic (apop) cells±10 μg PIC or 50 μg R848. Five days after immunization, mice were given PBSE-labelled target (OVA−or OVA+) cells. Twenty-four hours later, spleens were assessed for target cell frequency. Each dot represents one mouse. Data represent at least three independent experiments with 3–4 mice per group. **P<0.0015, *P<0.015,t-test. Indeed, IL-12 −/− IL-27 −/− mice did not display a suppressed CTL response beyond the effects observed in IL-27 −/− mice ( Fig 6c,d ). Although IL-12 production was selectively enhanced in the DC subsets stimulated by their corresponding TLR agonist, IL-27, and not IL-12, appears to be a key, but not sole, mediator for the induction of CTL against cell-associated and soluble antigens. Figure 6: IL-27 and not IL-12 is a key mediator for the induction of CTL. ( a ) DC subsets were isolated from PBS-perfused lung tissue for microarray analysis. Bars show relative mRNA expression of the indicated genes in pulmonary CD103 + DCs and CD11b + DCs treated± PIC or R848. ( b ) FACS analysis of migratory DCs isolated from LLN of IL-12p40 reporter mice, 24 h post i.n. instillation of 10 μg Poly I:C (PIC) or 50 μg R848. ( c , d ) OT-I CD8 T cells were adoptively transferred into WT, IL-12 −/− , IL-27 −/− or IL-12 −/− IL-27 −/− mice 1 day before i.n. delivery of PBS, sOVA or OVA + apoptotic (apop) cells±10 μg PIC or 50 μg R848. Five days after immunization, mice were given PBSE-labelled target (OVA − or OVA + ) cells. Twenty-four hours later, spleens were assessed for target cell frequency. Each dot represents one mouse. Data represent at least three independent experiments with 3–4 mice per group. ** P <0.0015, * P <0.015, t -test. Full size image Both CD103 + or CD11b + DCs can induce CTLs to prevent metastatic melanoma To confirm the initial experimental findings, we investigated in a metastatic melanoma model whether individual pulmonary DC subsets could induce endogenous melanoma-specific CTL (experimental outline, Supplementary Fig. 9a ). WT mice received two i.n. immunizations of apoptotic B16F10 melanoma cells with PBS, 10 μg Poly I:C or 50 μg R848, given 14 and 7 days before tumour challenge. Only CD103 + DCs trafficked apoptotic tumour cells to the LLNs ( Supplementary Fig. 9b ) [7] . Mice immunized with apoptotic B16F10 and Poly I:C (matched) showed nearly tumour-free lungs compared with the high tumour burden seen after immunization with PBS, apoptotic B16F10 alone, or apoptotic B16F10 with R848 (mismatched) ( Fig. 7a and Supplementary Fig. 9c ). Additional control mice were administered i.n. apoptotic B16F10 cells without i.v. B16F10 tumour challenge to confirm that the apoptotic tumour cells were themselves incapable of colonizing the lung ( Fig. 7a ). Consistent with the OVA model, CD103 + DCs required direct ligation of its PRR to induce endogenous tumour-specific CTL. 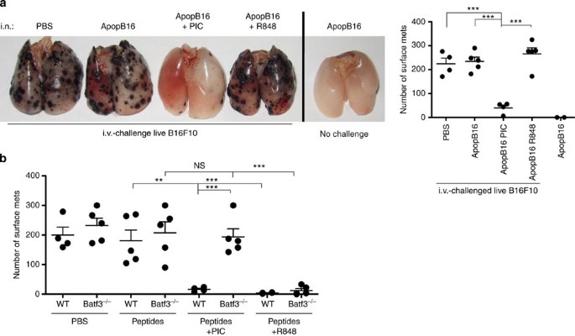Figure 7: Endogenous melanoma-specific CTLs are induced through the selective activation of antigen-bearing pulmonary DCs. (a) WT mice were delivered i.n. PBS or 10 × 106apoptotic (apop) B16F10±10 μg Poly I:C (PIC) or 50 μg R848, 14 and 7 days before an i.v. challenge of 2 × 105live B16F10 melanoma cells. WT mouse lungs were inflated 15 days after i.v. challenge. Control mice receive i.n. instillation of apoptotic B16F10 cells alone and were not given an i.v. challenge of live B16F10 cells. Samples were blinded and scored accordingly. Total surface metastases (mets) per lung were enumerated and shown by dot plots, each dot representing one mouse (right). Data are representative of three independent experiments with 4–5 mice per group. ***P<0.0001. (b) WT and Batf3−/−mice were delivered i.n PBS or 100 μg of each long tumour peptide PMEL, TRP-1 and TRP-2±10 μg PIC or 50 μg R848. Mice were immunized, challenged and scored as described above. Data are representative of three independent experiments with 4–5 mice per group. ***P<0.0001, **P<0.005,t-test. NS, non-significant. Figure 7: Endogenous melanoma-specific CTLs are induced through the selective activation of antigen-bearing pulmonary DCs. ( a ) WT mice were delivered i.n. PBS or 10 × 10 6 apoptotic (apop) B16F10±10 μg Poly I:C (PIC) or 50 μg R848, 14 and 7 days before an i.v. challenge of 2 × 10 5 live B16F10 melanoma cells. WT mouse lungs were inflated 15 days after i.v. challenge. Control mice receive i.n. instillation of apoptotic B16F10 cells alone and were not given an i.v. challenge of live B16F10 cells. Samples were blinded and scored accordingly. Total surface metastases (mets) per lung were enumerated and shown by dot plots, each dot representing one mouse (right). Data are representative of three independent experiments with 4–5 mice per group. *** P <0.0001. ( b ) WT and Batf3 −/− mice were delivered i.n PBS or 100 μg of each long tumour peptide PMEL, TRP-1 and TRP-2±10 μg PIC or 50 μg R848. Mice were immunized, challenged and scored as described above. Data are representative of three independent experiments with 4–5 mice per group. *** P <0.0001, ** P <0.005, t -test. NS, non-significant. Full size image Finally, the capacity for antigen-bearing CD11b + DCs to induce tumour-specific CTL was investigated. WT and Batf3 −/− mice received two immunizations of long tumour-specific peptides (PMEL, TRP-1 and TRP-2) with either PBS, 10 μg Poly I:C or 50 μg R848, 14 and 7 days before tumour challenge. Batf3 −/− mice, lacking CD103 + DCs, immunized with PBS, tumour-specific peptides alone or tumour-specific peptides with Poly I:C displayed similar numbers of surface tumours detected 16 days after tumour challenge ( Fig. 7b ). However, Batf3 −/− mice immunized with tumour-specific peptides and R848 were virtually tumour free. In control groups, WT mice immunized with tumour-specific peptides and Poly I:C or R848 also displayed virtually tumour-free lungs. Thus, CD11b + DCs are indeed able to induce endogenous tumour-specific CTL when stimulated by a TLR7 agonist. It is generally accepted that DC function is predetermined by lineage. Another possibility proposed in this study is that DC function is also determined by the nature of the PAMPs that stimulate it. Here, using a model antigen (OVA) and synthetic PAMP analogues instead of an infectious model (which usually generates more than one PAMP and antigenic form), we showed how individual DC subsets contribute to the induction of CTL. Specifically, we demonstrated that the induction of CTL only occurred when the antigen-bearing DC was activated through its corresponding PRR (matched, Supplementary Fig.1 ). Likewise, when the antigen-bearing DC was not directly stimulated through its PRR (mismatched, Supplementary Fig. 1 ), the outcome was CD8 T-cell proliferation but not a gain of cytotoxic function. This was further illustrated in a metastatic melanoma model lacking both the model antigen OVA and adoptively transferred OT-I T cells. In this scenario, only the proper activation of antigen-bearing CD103 + or CD11b + DCs provided protective immunity against the development of lung tumours, supporting the findings observed in the OVA model. The selectivity in DC subset activation likely restricts the inappropriate generation of CTL to bystander antigens created during inflammation. These findings build upon two elegant studies by Kratky et al. [14] and Sporri et al. [13] that demonstrated the need for direct TLR ligation on antigen-presenting cells to elicit T-cell immunity, which we now confirm, in vivo , at the endogenous DC subset level and extend this concept by demonstrating the required need to match antigen-bearing DCs with TLR agonists. Following the observation that matched versus mismatched DCs result in disparate T-cell-mediated immunity, we addressed whether the selective activation of CD103 + and CD11b + DCs with Poly I:C and R848, respectively, was mediated through TLR3 and TLR7. Consistent with previous studies, TLR3, an endosomal dsRNA sensor, was required for the induction of CTL when cell-associated antigens were immunized with Poly I:C [32] . In contrast, in the case of soluble antigen immunized with Poly I:C, both endosomal TLR3 and cytosolic dsRNA sensors appeared to be utilized. Only in the TLR3 −/− MAVS −/− mice, lacking both endosomal and cytosolic dsRNA-sensing pathways, was CTL induction prevented. One possible explanation for the variable DC activation in dsRNA-dependent pathways might be the difference between the uptake of apoptotic cells versus soluble proteins and its association with Poly I:C. Soluble antigens, such as OVA, may more readily gain access to the cytosol as demonstrated with cytochrome c ( Fig. 5b ). On the other hand, engulfed apoptotic cells are taken up into specialized endosomes (efferosomes) that may influence the processing of the engulfed antigen [38] . Apoptotic cells were mixed with Poly I:C minutes before immunization, which might have allowed the Poly I:C to settle onto the apoptotic cells and thus concentrating the dsRNA to apoptotic cell-containing endosomes, thereby limiting access to cytosolic sensors. In the future, it will be important to investigate how the nature of the antigen and PAMP drive antigen acquisition and processing by endogenous DC subsets. TLR7 ligation was required for the activation of CD11b + DCs to induce CTL. Examination of the CD11b + DCs in the absence of a TLR ligand, or with the non-cognate TLR3 stimulus Poly I:C, showed a correlative low, but distinct, ability to both cross-present and stimulate OT-I T cell replication, as well as to undergo a similar level of apoptosis in the presence of cytochrome c . CD11b + DCs that were stimulated with R848, but not with Poly I:C, underwent enhanced apoptosis in the presence of cytochrome c , ex vivo . Furthermore, activation of CD11b + DCs with R848 in vivo led to enhanced CD8 T-cell proliferation compared with CD11b + DCs exposed to Poly I:C. Thus, we conclude that the TLR7 stimulation of CD11b + DCs results in a marked increase of an inherent low-level ability to cross-present and an additional induction of the capacity to induce T-cell cytotoxicity via the production of the appropriate cytokines. To date, most studies assert lung CD103 + DCs as the ‘cross-presenting DCs’ versus the CD11b + DCs because this subset was shown to have a greater capacity to present exogenous proteins and cell-associated antigens to CD8 + T cells in steady state and during infection. Owing to their intrinsic antigen-presenting properties, CD103 + DCs have been regarded as the dominant DCs for antiviral immunity [4] , [5] , [17] , [21] , [23] , [39] , [40] , [41] . However, other studies have shown that pulmonary CD11b + DCs can elicit protective CD8 T-cell-mediated immunity against viral infections [42] . Therefore, the identity of the DC subset responsible in the induction of CTL during influenza infection remains controversial. This study may reconcile the differences in findings within the influenza literature. Using a reductionist approach, we demonstrated how individual DC subsets become activated and contribute to cytotoxic T-cell-mediated immunity. Through the engulfment of virus-infected cells, CD103 + DCs could recognize viral replication by TLR3 (ref. 32 ), or through the macropinocytosis of soluble factors along with replicating virus that could be translocated to the cytoplasm for dsRNA detection by dsRNA cytosolic sensors [33] , [43] . CD11b + DCs could detect viral infection via ssRNA engagement of TLR7 following the engulfment of cellular debris containing virus [44] . Thus, our study highlights potential mechanisms by which either CD103 + or CD11b + DCs might contribute to the development of T-cell-mediated immunity during an influenza infection. In addition to influenza, our findings may be relevant for cancer immunology. Ongoing clinical trials utilize TLR3 and TLR7 synthetic agonists, Poly IC:LC and Imiquimod, as adjuvants to activate DCs to generate strong tumour-specific T cells [45] . Both adjuvants have been shown to effectively stimulate DCs; however, which DC subset they selectively activate in humans remains unclear. In the future, it will be important to investigate how endogenous human DC subsets respond to TLR-based adjuvants. More recently, human DCs have been observed to display functional heterogeneity, similar to mice [46] , [47] , [48] , [49] , [50] , [51] , [52] , [53] . As human DC subsets are being characterized, it is apparent that disparity in PRR expression exists [48] , [54] . Observations, such as these, highlight the division of labour that exists among DC subsets and underscores the possibility of targeting human DC orthologues of the TLR3- and TLR7-expressing murine DCs to improve DC based vaccines against viruses and cancer. Mice CD45.1 and CD45.2 C57BL/6, 129/BL6 F2 (control for Batf3 −/− mice), OT-I, TLR3 −/− , TLR7 −/− , IL-12 −/− , IL-27 −/− , MDA5 −/− , MAVS −/− and C57BL/6-Tg(ACTB-OVA)916Jen/J mice were purchased from Jackson Research Laboratories and National Cancer Institute (NCI). CD45.1 OT-I, and TLR3 −/− MAVS −/− mice were bred in house. Batf3 −/− mice were kindly provided by Dr Kenneth Murphy. Mice were used for studies at 7–8 weeks of age, housed in a specific pathogen-free environment at National Jewish Health, an AAALAC accredited institution, and used in accordance with protocols approved by the Institutional Animal Care and Utilization Committee. Flow cytometry Single-cell suspensions were obtained from spleen, lungs and LLNs. All LLNs data were individually harvested (not pooled) for analysis. Before lung extraction, mice were perfused with 10 ml PBS. All tissues were minced and then digested with 2.5 mg ml −1 collagenase D (Roche) for 30 min at 37 °C. A quantity of 100 μl of 100 mM EDTA was added to stop 1 ml of enzymatic digestion. Digested tissue was pipetted up and down 30 times using a glass Pasteur pipette, and then passed through a 100-μm nylon filter to acquire single-cell suspensions. Spleens were treated with 7.5 ml of ammonium chloride lysing reagent (BD Biosciences), followed rapidly by the addition of 7.5 ml of Hanks' Balanced Salt Solution (HBSS). Cells were resuspended in fluorescence-activated cell sorting (FACS) blocking solution and stained at a 1/300 dilution for 30 min with conjugated antibodies obtained from Biolegend, eBioscience and BD Biosciences. The following purified monoclonal antibodies (mAbs) are used for staining: Pacific Blue (PB)-conjugated mAbs to CD8 and I-A/I-E; Phycoerythrin (PE)-conjugated mAbs to TLR3 and Siglec F; PerCP-Cy5.5- conjugated mAbs to CD4 or CD11b; PE-Cy7-conjugated mAb to CD11c; fluorescein isothiocyanate (FITC)-conjugated CD45.1 and CD45.2; allophycocyanin-Cy7-conjugated CD45 and Ly6C; and allophycocyanin-conjugated mAbs to CD103, EpCam, CD31 and CD45.1. Appropriate isotype-matched control mAbs were also obtained from eBioscience, BD Biosciences and Biolegend. F4/80-FITC was obtained from Serotec. Flow cytometry was performed using the LSR II (BD Biosciences) and data were analysed with FlowJo (Tree Star). Intracellular staining: following surface staining, cells were fixed and permeabilized using the Foxp3 staining buffer set and the provided protocol (eBioscience). Cells obtained from WT and TLR3 −/− mice were stained with PE-conjugated TLR3 (Biolegend). I.n. deliveries I.n. deliveries were performed using an optimized delivery system [27] , [55] . Mice were completely anaesthetized with avertin using 300 μl per mouse with tert -amyl alcohol content at 2.5% and 2,2,2 tribromoethanol (TCI America, T1420) at a concentration of 50 mg kg −1 . sOVA, apoptotic cells and TLR agonists were delivered in a 50 μl volume. Final concentration of deliveries were 1 μg sOVA (0.22 μ filtered, Grade VII Sigma) or 20 × 10 6 apoptotic cells±50 μg R848 (Enzo Life Sciences) or±10 μg Poly I:C (Enzo Life Sciences). Mice were killed at various times depending on the experimental design. Proliferation of OVA-specific transgenic CD8 + T cells Spleen cells from OT-I, in which the TCR of CD8 + cells are restricted to OVA, were isolated and labelled with 10 μM CFSE. Half a million of these cells were transferred i.v. into recipient mice 1 day before i.n. delivery of apoptotic cells and sOVA. Mice were killed 3 days after i.n. deliveries for analysis of T-cell proliferation (CFSE dye dilution) in the LLN. For intracellular cytokine staining, LLNs were isolated 3 days after i.n. deliveries of apoptotic cells or sOVA±Poly I:C and digested in collagenase D for 30 min, then pressed through a 100-μm nylon filter to obtain single-cell suspensions of antigen-presenting cells and proliferating T cells. Isolated cells were cultured 5 h in RPMI-10% fetal calf serum (FCS) containing 10 μM OVA peptide (257–264) and Brefeldin A 10 μg ml −1 . Following surface staining, BD Foxp3 intracellular staining kit was used. Cells were stained with allophycocyanin (APC)-conjugated to IFNγ, PerCP-Cy5.5-TNFα, PECy7-granzymeB or isotype controls (BD Pharmingen). Proliferation of endogenous OVA-specific CD8 + T cells Mice were delivered 100 μg sOVA (0.22 μ filtered, Grade VII Sigma)±100 μg Poly I:C (Enzo Life Sciences). Four days later, LLN were harvested for H-2Kb/SIINFEKL tetramer staining (Beckman Coulter) for flow analysis. Cytochrome c assay Pulmonary CD11c + cells were enriched by positive selection using CD11c + MicroBeads (Miltenyi Biotec). CD11c + cells (100,000) per well were plated in 96-well plates overnight in RPMI-10% FCS with or without 10 mg ml −1 horse cytochrome c (Sigma), along with PBS, 10 μg ml −1 Poly I:C or 50 μg ml −1 R848. In vivo cytotoxic T-cell assay First, we performed a dose-dependent analysis of OT-I T-cell proliferation response to Poly I:C and R848. An amount of 10 μg for Poly I:C and 50 μg for R848 were selected based on their capacity to induce quantitatively similar OT-I T-cell proliferation ( Supplementary Fig. 10 ). One day after OT-I cell adoptive transfer, WT mice were administered by i.n. delivery with 1 μg sOVA (0.22 μ filtered, Grade VII Sigma) WT-apoptotic or OVA-apoptotic cells±10 μg Poly I:C (Enzo Life Sciences) or 50 μg R848 (Enzo Life Sciences). Five days after immunization, in vivo target cells were labelled using 15 μM PBSE. A quantity of 10 7 PBSE-labelled CD45.1 WT and CD45.2 OVA-expressing splenocytes (derived from ACTB-OVA mice) were injected at a (1:1) ratio i.v. The following day, spleens were harvested as described and specific killing of adoptively transferred congenic mismatched populations was assessed by flow cytometry. Anti-Gr1 monocyte and plasmacytoid DC depletion To deplete monocytes and plasmacytoid DCs, 400 μg anti-mouse Ly-6G (Gr1) functional-grade purified antibody (eBioscience) or Rat IgG2b isotype control was injected into the peritoneal cavity 24 h before i.n. immunizations. Blood, spleen, LLN and lung were taken at 24 h to assess cellular depletion. CD45.1 OT-I T-cell transfer CD45.1 OT-I T cells were transferred into eight CD45.2 WT or 10 CD45.2 Batf3 −/− followed by i.n. immunization with 1 μg sOVA (0.22 μ filtered, Grade VII Sigma)+10 μg Poly I:C. Five days after immunization, CD45.1 OT-I T cells were positively selected from the spleens of WT and Batf3 −/− mice using biotinylated anti-CD45.1 antibody (eBioscience) and anti-biotin MicroBeads (Miltenyi Biotec). CD45.1 OT-I T cells (1 × 10 6 ) differentiated in WT or Batf3 −/− mice were transferred into naive C57BL/6 hosts. Twenty-four hours after CD45.1 OT-I T-cell transfer, (1:1) OVA + (OVA expressing) and OVA − (WT) target cells were transferred. Twenty-four hours after target cell transfer, spleens were harvested for the analysis of target cell killing. Type I IFN detection Whole lungs of WT and Batf3 −/− mice were homogenized using a tissue homogenizer 10 h after i.n. deliver of 10 μg Poly I:C or PBS in a 50-μl volume. Supernatants were collected, and IFNβ and IFNα concentrations were determined by enzyme-linked immunosorbent assay (R&D Systems). Microscopy CFSE-labelled apoptotic cells and 1 μg sOVA-Alexa-647, or sOVA-FITC were co-delivered i.n. with 5 μg rhodamine-labelled Poly I:C (Invivogen). Two hours post delivery, lungs were digested, and CD103 + DCs were isolated using biotinylated anti-CD103 antibody (eBioscience) and anti-biotin MicroBeads (Miltenyi Biotec). Cells were then cytospun, mounted with 4',6-diamidino-2-phenylindole (DAPI) and imaged using a Leica confocal microscope. Apoptotic cell delivery Thymocytes were obtained from C57BL/6 and ACTB-OVA mice 7–8 weeks of age. Single-cell suspensions were made using the rubber end of a syringe and mashing cells through a 40-μm nylon filter. Apoptosis of murine thymocytes was induced by 60 mJ UV radiation exposure (Stratagene 1800 StrataLinker). Apoptosis of B16F10 tumour cells was induced with 100 Gy using a Gamma cell irradiator. Phosphatidylserine exposure was detected by Annexin V staining and propidium iodide to assure that no necrotic cells were present before delivery. CFSE-labelled apoptotic B16F10 cells trafficked by DCs were assessed in the LLN 24 h after delivery into the lungs by flow cytometry [7] . B16F10 melanoma model for lung metastasis B16F10 melanoma cells, kindly provided by Drs Ross Kedl and Jill Slansky, were maintained in RPMI +10% FCS supplemented with 1% Pen/Strep/ L -glutamine (Sigma), 1% non-essential amino acids (Sigma), 1% sodium pyruvate (Sigma), 10 mM HEPES (Sigma) and 0.1 mM β-mercaptoethanol. Mice were immunized i.n. with apoptotic B16F10 melanoma cells or long tumour peptides of PMEL, TRP-1 and TRP-2±10 μg Poly I:C, 50 μg R848 or PBS 14 days and 7 days before i.v. challenge with 2 × 10 5 viable B16F10 cells. Mice were euthanized 15 days after i.v. tumour challenge. Lungs of mice were inflated with 1% agarose. Two blinded observers counted the B16F10 metastases. Gene array Whole-mouse genome Affymetrix gene arrays were performed with the Immunological Genome Project (ImmGen) at Harvard University [56] . As per the specifications of ImmGen, we followed a standard operation procedure for the isolation and purification of all cell populations that is uniform across the ImmGen data set. Procedures for cell isolation, sorting and RNA extractions are outlined in extensive detail at www.immgen.org . PBS-perfused treated and untreated lungs were digested using 1.75 mg ml −1 Liberase blendzyme 3 (Roche) for 15 min, filtered two times through 100 μm nylon strainer, washed with HBSS and then stained with conjugated flow cytometry antibodies (eBioscience) to identify pulmonary DCs. Propidium iodide was used to exclude dead cells. Cell populations were sorted twice to enhance purity (BD Aria). The entire procedure from the time of killing to cells collected in Trizol was completed in <3 h, a requirement by ImmGen. Flow plots of the actual sorts and cells used for RNA extraction may be viewed at www.immgen.org . All data sets have been deposited at National Center for Biotechnology Information/Gene Expression Omnibus under accession number GSE15907 . Statistics Statistical analysis was conducted using InStat and Prism software (both from GraphPad). All results are expressed as the mean±s.e.m. Statistical tests were performed using two-tailed Student’s t -test. A value of P <0.05 was considered statistically significant. How to cite this article: Desch, AN. et al. Dendritic cell subsets require cis-activation for cytotoxic CD8 T-cell induction. Nat. Commun. 5:4674 doi: 10.1038/ncomms5674 (2014).